Robust photoregulation of GABAAreceptors by allosteric modulation with a propofol analogue Photochemical switches represent a powerful method for improving pharmacological therapies and controlling cellular physiology. Here we report the photoregulation of GABA A receptors (GABA A Rs) by a derivative of propofol (2,6-diisopropylphenol), a GABA A R allosteric modulator, which we have modified to contain photoisomerizable azobenzene. Using α 1 β 2 γ 2 GABA A Rs expressed in Xenopus laevis oocytes and native GABA A Rs of isolated retinal ganglion cells, we show that the trans -azobenzene isomer of the new compound ( trans - MPC088 ), generated by visible light (wavelengths ~440 nm), potentiates the γ-aminobutyric acid-elicited response and, at higher concentrations, directly activates the receptors. cis -MPC088, generated from trans - MPC088 by ultraviolet light (~365 nm), produces little, if any, receptor potentiation/activation. In cerebellar slices, MPC088 co-applied with γ-aminobutyric acid affords bidirectional photomodulation of Purkinje cell membrane current and spike-firing rate. The findings demonstrate photocontrol of GABA A Rs by an allosteric ligand, and open new avenues for fundamental and clinically oriented research on GABA A Rs, a major class of neurotransmitter receptors in the central nervous system. Synthetically modifying the neurotransmitter agonist of a postsynaptic receptor to contain a chemical photoswitch has been shown to afford photocontrol of ionotropic receptors for acetylcholine and L -glutamate through regulation of the access of the neurotransmitter moiety to its binding site [1] , [2] . A different approach is to engineer photoregulation through a modulator rather than an agonist, by perturbing the receptor structure at a site distinct from the neurotransmitter-binding pocket. The abundance and diversity of known allosteric modulators of receptor proteins suggest the feasibility of this alternative approach. Given that receptor modulators typically act in concert with endogenous signals in a neural network, a photoswitchable modulator could potentially enable relatively subtle conditional control of neuronal excitability. GABA A receptors (GABA A Rs) are pentameric ligand-gated ion channels that function as postsynaptic and extrasynaptic receptors for the inhibitory neurotransmitter γ-aminobutyric acid (GABA) in the brain and retina [3] , [4] , [5] . The α 1 β 2 γ 2 GABA A R, which consists of two α 1 subunits, two β 2 subunits and a single γ 2 subunit, is among the most abundant and widely distributed of this receptor type. A number of naturally occurring and synthetic low-molecular weight compounds are known to modulate the α 1 β 2 γ 2 GABA A R response to GABA [3] . Among the most extensively studied GABA A R modulators is propofol ( Fig. 1a ), a non-volatile anaesthetic that allosterically potentiates the GABA response and, at high concentrations, directly activates the receptor [6] , [7] , [8] , [9] , [10] , [11] , [12] . Behavioural studies indicate that propofol exerts its anaesthetic actions by modulating GABA A Rs [13] , [14] . With the aim of developing photoregulated GABA A R-directed ligands, we have investigated propofol derivatives that contain azobenzene, a widely studied photoisomerizable chemical residue capable of bidirectional switching between trans - and cis -geometrical isomers [1] , [2] , [15] , [16] , [17] , [18] , [19] , [20] . Here we describe the development of a compound, termed MPC088 ( Fig. 1a ), which displays robust light-regulated activity at GABA A Rs. To our knowledge, the present study is the first to report photocontrol of a neurotransmitter receptor by a cis–trans photoisomerizable compound derived from an allosteric ligand. The findings establish a new modality by which to regulate GABA A Rs, a receptor type of major importance to central nervous system (CNS) function. 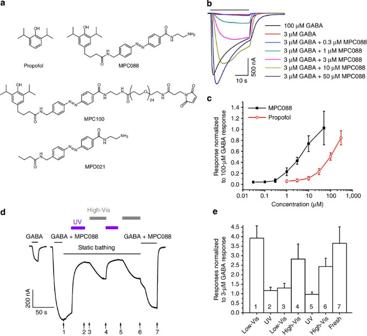Figure 1: Effect ofMPC088on the 3 μM GABA response of α1β2γ2GABAAR-expressing oocytes. (a) Chemical structures. (b) Responses of a single oocyte to co-applied 3 μM GABA and varying concentration oftrans-dominantMPC088. Horizontal bar indicates the period of superfusion with GABA- andMPC088-supplemented Ringer solution. (c) Aggregate concentration–response data (mean±s.d.) describing responses elicited by co-applied 3 μM GABA andtrans-dominantMPC088or propofol. Response amplitudes obtained from each oocyte normalized to that elicited by 100 μM GABA alone, a near-saturating condition that is essentially insensitive to propofol potentiation.MPC088and propofol results, each obtained from seven oocytes. (d) Light-dependent alteration of the 3-μM GABA response by co-applied, initiallytrans-dominant, 1 μMMPC088. Black bars: periods of superfusion with co-applied 3 μM GABA and 1 μMMPC088. Purple and grey bars: period of presentation of ultraviolet (UV) light and high-intensity visible light (High-Vis), respectively. (e) Results obtained in the experiment ofdand three others of similar design (mean±s.d.). Membrane current amplitudes, normalized to the peak amplitude of the 3-μM GABA response, determined under seven sequential conditions: (1) in low-intensity visible light (Low-Vis), at the conclusion of superfusion with (3 μM GABA+1 μMMPC088); (2) at the conclusion of UV illumination; (3) in Low-Vis; (4) at the conclusion of high-intensity visible illumination; (5) at the conclusion of a second UV illumination; (6) at the conclusion of a second high-intensity visible illumination; and (7) at the conclusion of resumed superfusion with fresh 3 μM GABA+1 μMtrans-dominantMPC088. These amplitude determination conditions are denoted by numbers beneath the waveform ind. Repeated-measures analysis of variance conducted on the aggregate data yieldedF(6,18)=41.975,P<0.001.Post-hocpaired-sample Student'st-tests corrected for multiple comparisons indicated significant differences produced by the initial UV, the initial High-Vis, the second UV, and the second High-Vis illuminations (P≤0.009 for amplitude group 2 versus group 1, for 4 versus 3, for 5 versus 4, and for 6 versus 5, respectively); amplitude groups 7 and 1 did not differ significantly (P=0.075). Figure 1: Effect of MPC088 on the 3 μM GABA response of α 1 β 2 γ 2 GABA A R-expressing oocytes. ( a ) Chemical structures. ( b ) Responses of a single oocyte to co-applied 3 μM GABA and varying concentration of trans -dominant MPC088 . Horizontal bar indicates the period of superfusion with GABA- and MPC088 -supplemented Ringer solution. ( c ) Aggregate concentration–response data (mean±s.d.) describing responses elicited by co-applied 3 μM GABA and trans -dominant MPC088 or propofol. Response amplitudes obtained from each oocyte normalized to that elicited by 100 μM GABA alone, a near-saturating condition that is essentially insensitive to propofol potentiation. MPC088 and propofol results, each obtained from seven oocytes. ( d ) Light-dependent alteration of the 3-μM GABA response by co-applied, initially trans -dominant, 1 μM MPC088 . Black bars: periods of superfusion with co-applied 3 μM GABA and 1 μM MPC088 . Purple and grey bars: period of presentation of ultraviolet (UV) light and high-intensity visible light (High-Vis), respectively. ( e ) Results obtained in the experiment of d and three others of similar design (mean±s.d.). Membrane current amplitudes, normalized to the peak amplitude of the 3-μM GABA response, determined under seven sequential conditions: (1) in low-intensity visible light (Low-Vis), at the conclusion of superfusion with (3 μM GABA+1 μM MPC088 ); (2) at the conclusion of UV illumination; (3) in Low-Vis; (4) at the conclusion of high-intensity visible illumination; (5) at the conclusion of a second UV illumination; (6) at the conclusion of a second high-intensity visible illumination; and (7) at the conclusion of resumed superfusion with fresh 3 μM GABA+1 μM trans -dominant MPC088 . These amplitude determination conditions are denoted by numbers beneath the waveform in d . Repeated-measures analysis of variance conducted on the aggregate data yielded F (6,18)=41.975, P <0.001. Post-hoc paired-sample Student's t -tests corrected for multiple comparisons indicated significant differences produced by the initial UV, the initial High-Vis, the second UV, and the second High-Vis illuminations ( P ≤0.009 for amplitude group 2 versus group 1, for 4 versus 3, for 5 versus 4, and for 6 versus 5, respectively); amplitude groups 7 and 1 did not differ significantly ( P =0.075). Full size image Light-regulated potentiation of α 1 β 2 γ 2 GABA A R activity Chemical synthesis and purification yielded MPC088 preparations consisting of the trans - and cis -isomers in proportions that were trans -dominant (typically, about 95%; Supplementary Methods ). Spectrophotometric and NMR data indicated that, as with unmodified azobenzene, ultraviolet (UV) light (wavelengths near 365 nm) isomerizes the trans -isomer of MPC088 to the cis form, which is stable for many hours in darkness, and visible (or blue) light (containing wavelengths near 440 nm) drives the cis - to trans -isomerization ( Supplementary Note 1 and Supplementary Figs S1–S2 ). In Xenopus oocytes expressing α 1 β 2 γ 2 GABA A Rs, 3 μM GABA elicits a response ~4–10% of the saturation level, and was used to test for response enhancement by MPC088 . When co-applied with 3 μM GABA, MPC088 in predominantly the trans -isomer form increased the response in a concentration-dependent fashion ( Fig. 1b ) and exhibited a potency ~25 times that of propofol, as determined by the relationship of the MPC088 versus propofol concentration for which the peak response amplitude was 50% of that elicited by 100 μM GABA alone ( Fig. 1c ). By analogy with the known effects of propofol, this action of MPC088 could reflect contributions from both potentiation of the GABA response and direct receptor activation (that is, direct agonist activity). We tested for potentiation by MPC088 at a concentration (1 μM) associated with negligible direct activation, and specifically investigated the effect of light that isomerizes the azobenzene moiety ( Fig. 1d,e ). Co-applied 3 μM GABA and 1 μM trans -dominant MPC088 markedly potentiated the GABA response, and brief UV illumination presented during static bathing of the oocyte decreased the membrane current to a level near that elicited by GABA alone ( Supplementary Note 2 ). This level of current was maintained in the ambient light after cessation of the UV illumination and, conversely, was increased by exposure to high-intensity visible light. The resumption of perfusion with co-applied GABA and trans -dominant MPC088 restored the membrane current to a level near that exhibited on initial presentation of the two compounds. By contrast, MPD021 ( Fig. 1a ) that lacks the propofol moiety showed no potentiation of the GABA response and failed to inhibit potentiation by MPC088 ( Supplementary Note 3 ). Light-regulated direct activation of α 1 β 2 γ 2 GABA A Rs In addition to potentiation, trans -dominant MPC088 robustly activated α 1 β 2 γ 2 GABA A Rs ( Fig. 2 ). The response elicited by trans -dominant MPC088 was graded with concentration, evident at concentrations as low as 4 μM ( Fig. 2a,b ), and greater than the response to a matched concentration of cis -dominant MPC088. The maximum current generated by trans -dominant MPC088 was comparable to the peak current elicited by 100 μM GABA, whereas that generated by propofol represented only about 40% of the 100 μM GABA response. The potency of trans -dominant MPC088 exceeded that of propofol by ~25-fold, as determined by the concentrations of MPC088 versus propofol required for a peak current equal to 40% of the 100 μM GABA-alone response ( Fig. 2b ). The MPC088 -elicited response was eliminated by the GABA A R channel blocker picrotoxin (PTX) [21] , but was not sensitive to gabazine (SR-95531)—a competitive GABA antagonist [22] , [23] —and was only partially antagonized by bicuculline [8] , [24] ( Fig. 2b inset). These properties, which are shared by the known GABA A R allosteric activators alphaxalone [10] , [22] and pentobarbital [24] , [25] , suggested that MPC088 activates the receptors by binding at a site distinct from the GABA-binding site. UV illumination presented during static bathing reduced the MPC088 -elicited current, and visible light reversed the effect of UV exposure ( Fig. 2c,d ). Furthermore, repeated pulses of UV light presented on a background of continuous visible light during MPC088 treatment yielded cyclic changes in response amplitude ( Fig. 2e ). Together, the data of Figs 1 and 2 do not rule out an action of cis MPC088 in receptor potentiation or direct activation ( Supplementary Note 4 ), but indicate that any such activity is much weaker than that of the trans -isomer. 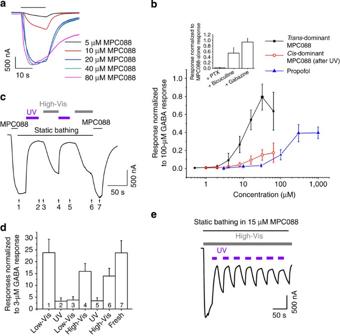Figure 2:MPC088agonist activity in oocytes expressing α1β2γ2GABAARs. (a) Representative responses toMPC088obtained in a single experiment. (b) Concentration–response functions (mean±s.d.) fortrans- andcis-dominant MPC088 (n=6) and propofol (n=6). In each of theMPC088experiments, thecis-dominant form was generated by UV light during static bathing. Amplitudes normalized to the 100-μM GABA response. Inset: sensitivity (mean±s.d.) of theMPC088(15 μM) response to 100 μM PTX (n=4), 100 μM bicuculline (n=4) and 30 μM gabazine (n=4). (c) Photoregulation of the response to 15 μMMPC088. (d) Normalized current amplitudes (mean±s.d.) determined in the experiment ofcand in three others of similar design. Amplitudes in each experiment normalized to that elicited by 3 μM GABA. Numbers beneath the waveform incdenote amplitude determination conditions for the experiment shown inc. Repeated-measures analysis of variance conducted on the aggregate data yieldedF(6,18)=68.988,P<0.001.Post-hocpaired-sample Student'st-tests corrected for multiple comparisons indicated significant differences produced by the initial UV, the initial high-intensity visible light (High-Vis), the second UV, and the second High-Vis illuminations (P≤0.010 for amplitude group 2 versus group 1, for 4 versus 3, for 5 versus 4, and for 6 versus 5, respectively); amplitude groups 7 and 1 did not differ significantly (P=0.96). (e) Representative waveform obtained with repeated presentation of UV light during continuous High-Vis illumination (static bathing inMPC088-supplemented Ringer). Figure 2: MPC088 agonist activity in oocytes expressing α 1 β 2 γ 2 GABA A Rs. ( a ) Representative responses to MPC088 obtained in a single experiment. ( b ) Concentration–response functions (mean±s.d.) for trans - and cis -dominant MPC088 ( n =6) and propofol ( n =6). In each of the MPC088 experiments, the cis -dominant form was generated by UV light during static bathing. Amplitudes normalized to the 100-μM GABA response. Inset: sensitivity (mean±s.d.) of the MPC088 (15 μM) response to 100 μM PTX ( n =4), 100 μM bicuculline ( n =4) and 30 μM gabazine ( n =4). ( c ) Photoregulation of the response to 15 μM MPC088 . ( d ) Normalized current amplitudes (mean±s.d.) determined in the experiment of c and in three others of similar design. Amplitudes in each experiment normalized to that elicited by 3 μM GABA. Numbers beneath the waveform in c denote amplitude determination conditions for the experiment shown in c . Repeated-measures analysis of variance conducted on the aggregate data yielded F (6,18)=68.988, P <0.001. Post-hoc paired-sample Student's t -tests corrected for multiple comparisons indicated significant differences produced by the initial UV, the initial high-intensity visible light (High-Vis), the second UV, and the second High-Vis illuminations ( P ≤0.010 for amplitude group 2 versus group 1, for 4 versus 3, for 5 versus 4, and for 6 versus 5, respectively); amplitude groups 7 and 1 did not differ significantly ( P =0.96). ( e ) Representative waveform obtained with repeated presentation of UV light during continuous High-Vis illumination (static bathing in MPC088 -supplemented Ringer). Full size image Activity at GABA A Rs of differing subunit composition Propofol is known to modulate GABA A Rs that contain a β-subunit. To determine whether trans - MPC088 is active at other β-containing GABA A R subtypes, we tested the compound in oocytes expressing α 1 β 3 γ 2 , a GABA A R that, like α 1 β 2 γ 2 , is widely expressed in CNS neurons [3] , [26] , [27] , [28] , and α 4 β 3 δ, a subtype that is typically expressed extrasynaptically and exhibits high sensitivity to GABA [3] , [5] , [29] . Trans -dominant MPC088 showed potentiating activity on both receptor types ( Fig. 3a ), and this activity was reduced by UV illumination (not shown). With co-applied 3 μM GABA (representing ~EC 8 ), the α 1 β 3 γ 2 GABA A R response function obtained with trans -dominant MPC088 closely resembled the response function determined for the α 1 β 2 γ 2 subtype. By contrast, the trans - MPC088 response function obtained for α 4 β 3 δ with co-applied 50 nM GABA (~EC 8 ) approached a plateau representing ~42% of the response amplitude obtained with high GABA concentration. The low plateau level of the α 4 β 3 δ response to trans - MPC088 did not reflect a general insensitivity to propofol-based compounds, as co-applied 200 μM propofol and 50 nM GABA yielded a response representing 1.2±0.1-fold ( n =4) that of the saturating GABA-alone response. In addition, the direct agonist activity of trans - MPC088 at α 4 β 3 δ was much lower than those at α 1 β 3 γ 2 and α 1 β 2 γ 2 ( Fig. 3b ). Thus, trans - MPC088 , like propofol, modulates multiple types of β-containing GABA A Rs, albeit with different efficacy. We also tested the activity of trans -dominant MPC088 at receptors containing the β-subunit substitution N265M, a mutation that markedly reduces the action of propofol both in vitro and in vivo [13] , [30] . These experiments specifically involved comparison of the normalized responses of α 1 β 3 γ 2 and α 1 β 3 (N265M)γ 2 GABA A Rs to trans - MPC088 (1 μM) and co-applied GABA. Response enhancement by trans - MPC088 was substantial at both receptor types, but that for α 1 β 3 (N265M)γ 2 (2.9±0.8-fold, n =4) was significantly smaller than that for the wild-type α 1 β 3 γ 2 (4.4±1.3-fold, n =5; P =0.03, two-sample Student's t -test; Supplementary Fig. S3 ). Like propofol, trans - MPC088 lacked both potentiating and direct agonist activity on oocytes expressing the GABA A R subtype that consists of a pentameric assembly of ρ1 subunits [31] . 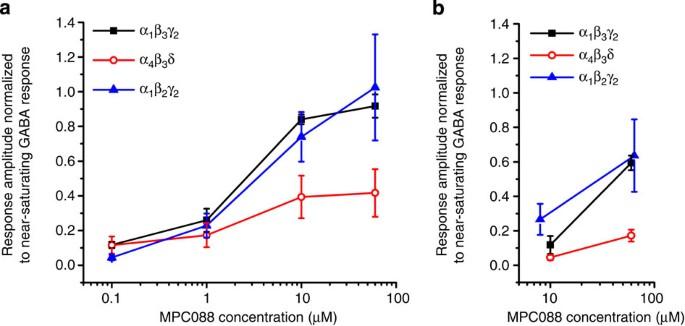Figure 3: Effect ofMPC088on α1β3γ2and α4β3δ GABAAR-expressing oocytes. Data in each group obtained from four oocytes. (a) Aggregate concentration–response data (mean±s.d.) obtained from α1β3γ2(black) and α4β3δ (red) receptors with co-applied GABA at similar ~EC8dose (that is, 3 μM for the former and 0.05 μM for the latter receptor type) and varying concentrations oftrans-dominantMPC088. Response amplitudes obtained from each oocyte normalized to its saturating GABA response (that is, responses obtained with 1,000 μM GABA for α1β3γ2and 100 μM GABA for α4β3δ GABAARs). (b) Aggregate concentration–response data (mean±s.d.) obtained from α1β3γ2(black) and α4β3δ (red) receptors withtrans-dominantMPC088alone. Data similarly normalized to the saturating GABA response obtained from each oocyte. Results for α1β2γ2GABAARs inaandb(blue) reproduced from those ofFigs 1cand2b, respectively. Figure 3: Effect of MPC088 on α 1 β 3 γ 2 and α 4 β 3 δ GABA A R-expressing oocytes. Data in each group obtained from four oocytes. ( a ) Aggregate concentration–response data (mean±s.d.) obtained from α 1 β 3 γ 2 (black) and α 4 β 3 δ (red) receptors with co-applied GABA at similar ~EC 8 dose (that is, 3 μM for the former and 0.05 μM for the latter receptor type) and varying concentrations of trans -dominant MPC088 . Response amplitudes obtained from each oocyte normalized to its saturating GABA response (that is, responses obtained with 1,000 μM GABA for α 1 β 3 γ 2 and 100 μM GABA for α 4 β 3 δ GABA A Rs). ( b ) Aggregate concentration–response data (mean±s.d.) obtained from α 1 β 3 γ 2 (black) and α 4 β 3 δ (red) receptors with trans -dominant MPC088 alone. Data similarly normalized to the saturating GABA response obtained from each oocyte. Results for α 1 β 2 γ 2 GABA A Rs in a and b (blue) reproduced from those of Figs 1c and 2b , respectively. Full size image Receptor-tethered MPC088 analogue MPC088 is a freely diffusible compound and can be removed by superfusion of the oocyte with Ringer. We asked whether covalent tethering of a similar compound to a suitably modified receptor produces persistent potentiation and/or activation. MPC100 ( Fig. 1a ), prepared by coupling a maleimide-terminated 24-mer poly(ethylene glycol) (PEG) linker to the free amino group of MPC088 , was tested on oocytes expressing a cysteine substitution at position 79 of the single γ-subunit of α 1 β 2 γ 2 [α 1 β 2 γ 2 (A79C)] [32] , [33] , abbreviated as γ-79C. The thiol group of the cysteine residue allowed covalent anchoring of MPC100 (refs 15 , 17 , 19 ). Oocytes expressing γ-79C GABA A Rs, following incubation with trans -dominant MPC100 and then superfusion with unsupplemented Ringer to remove untethered compound, exhibited persistent potentiation of the GABA response ( Fig. 4a,b ), which was sensitive to UV and visible light ( Fig. 4c ). These effects of illumination resembled those displayed by wild-type α 1 β 2 γ 2 GABA A R-expressing oocytes in the presence of co-applied GABA and MPC088 (compare Figs 1d and 4c ), although the extent of UV-induced depotentiation observed with the tethered MPC100 was less than that determined on similar treatment with (diffusible) MPC088 . The smaller excursion of depotentiation likely resulted from the inability of the UV-stimulating light, which was delivered from above the (opaque) oocyte, to efficiently access MPC100 tethered to the lower, approximately hemispherical surface of the cell. 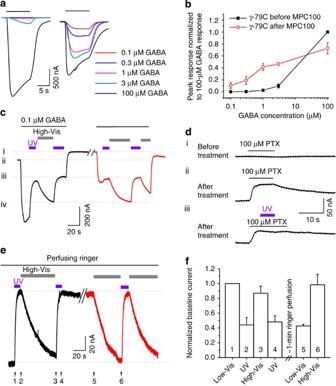Figure 4: Persistent potentiation and activation byMPC100in γ-79C-expressing oocytes. (a) GABA responses of a single oocyte before (left) and after (right)MPC100treatment (100 μM). Right-hand waveforms recorded after ~7-min incubation withMPC100and subsequent Ringer perfusion. (b) GABA response functions showing aggregate data (mean±s.d.; five oocytes) obtained beforeMPC100treatment, and after treatment with 100 μMMPC100and subsequent washout (~5 min). Amplitudes normalized to that elicited by 100 μM GABA beforeMPC100treatment. (c) Light-dependence of persistent potentiation. Black trace: response to UV and visible light in the presence of 0.1 μM GABA, following treatment with 100 μMtrans-dominantMPC100. Dotted lines i and ii highlight the difference in baseline current before (ii) versus after (i) UV illumination). Red trace: later phase of the same experiment (responses obtained after a further ~1 min Ringer perfusion). (d) Baseline currents obtained in a single experiment. Trace i: nominal response to PTX (100 μM). Traces ii, iii: PTX responses obtained after treatment with 100 μMMPC100in the absence (ii) and presence (iii) of UV illumination. (e) Responses to UV and visible light following exposure totrans-dominantMPC100and washout (~5 min) of freeMPC100. Data obtained from a single oocyte. A period of Ringer perfusion (~1 min) separated the initial (black trace) and later (red trace) phases of the experiment. (f) Aggregate results (mean±s.d.) from experimenteand three others, each involving amplitude determinations under six sequential experimental conditions. Data normalized to the persisting shift in baseline produced byMPC100treatment. Periods of treatment in each experiment were similar to those illustrated ine. Numbers beneath the waveforms inedenote amplitude determination conditions for the experiment shown ine. Repeated-measures analysis of variance conducted on the aggregate data yieldedF(6,18)=65.290,P<0.001.Post-hocpaired-sample Student'st-tests corrected for multiple comparisons indicated significant differences produced by the initial UV, the initial high-intensity visible light (High-Vis), the second UV, and the second High-Vis illuminations (P≤0.007 for amplitude group 2 versus group 1, for 3 versus 2, for 4 versus 3, and for 6 versus 5, respectively). Figure 4: Persistent potentiation and activation by MPC100 in γ-79C-expressing oocytes. ( a ) GABA responses of a single oocyte before (left) and after (right) MPC100 treatment (100 μM). Right-hand waveforms recorded after ~7-min incubation with MPC100 and subsequent Ringer perfusion. ( b ) GABA response functions showing aggregate data (mean±s.d. ; five oocytes) obtained before MPC100 treatment, and after treatment with 100 μM MPC100 and subsequent washout (~5 min). Amplitudes normalized to that elicited by 100 μM GABA before MPC100 treatment. ( c ) Light-dependence of persistent potentiation. Black trace: response to UV and visible light in the presence of 0.1 μM GABA, following treatment with 100 μM trans -dominant MPC100 . Dotted lines i and ii highlight the difference in baseline current before (ii) versus after (i) UV illumination). Red trace: later phase of the same experiment (responses obtained after a further ~1 min Ringer perfusion). ( d ) Baseline currents obtained in a single experiment. Trace i: nominal response to PTX (100 μM). Traces ii, iii: PTX responses obtained after treatment with 100 μM MPC100 in the absence (ii) and presence (iii) of UV illumination. ( e ) Responses to UV and visible light following exposure to trans -dominant MPC100 and washout (~5 min) of free MPC100 . Data obtained from a single oocyte. A period of Ringer perfusion (~1 min) separated the initial (black trace) and later (red trace) phases of the experiment. ( f ) Aggregate results (mean±s.d.) from experiment e and three others, each involving amplitude determinations under six sequential experimental conditions. Data normalized to the persisting shift in baseline produced by MPC100 treatment. Periods of treatment in each experiment were similar to those illustrated in e . Numbers beneath the waveforms in e denote amplitude determination conditions for the experiment shown in e . Repeated-measures analysis of variance conducted on the aggregate data yielded F (6,18)=65.290, P <0.001. Post-hoc paired-sample Student's t -tests corrected for multiple comparisons indicated significant differences produced by the initial UV, the initial high-intensity visible light (High-Vis), the second UV, and the second High-Vis illuminations ( P ≤0.007 for amplitude group 2 versus group 1, for 3 versus 2, for 4 versus 3, and for 6 versus 5, respectively). Full size image Treatment of γ-79C-expressing oocytes with trans -dominant MPC100 led to a greater (that is, more negative) baseline current, and UV illumination produced an opposite change ( Fig. 4c ; note the relationship of the dotted reference lines i and ii). To test whether the baseline change reflected continuing, direct activation by the tethered MPC100 in the absence of GABA, we investigated the effect of PTX presented before and after MPC100 treatment. PTX application to MPC100 -treated and then washed cells reversibly reduced the baseline current by 85±7% ( n =5; Fig. 4d , traces i–ii). UV (that is, cis -generating) illumination delivered during PTX treatment did not further reduce the baseline amplitude, but inhibited baseline recovery following PTX removal, consistent with a UV-induced reduction in the amount of trans - MPC100 present ( Fig. 4d , trace iii). Furthermore, UV and visible light delivered to MPC100 -treated γ-79C-expressing oocytes produced, respectively, decreases and increases in membrane current, qualitatively similar to those exhibited by wild-type α 1 β 2 γ 2 GABA A Rs in the presence of trans - MPC088 alone ( Fig. 4e,f ). Thus, the larger baseline current persisting after MPC100 treatment ( Fig. 4c ) reflected sustained, direct activation of the receptor by tethered trans - MPC100 . These persistent effects of MPC100 required the γ-79C modification. Although MPC100 exhibited potentiation on wild-type α 1 β 2 γ 2 GABA A Rs (albeit to an extent less than that exhibited by MPC088 ), this effect was eliminated by Ringer perfusion ( Supplementary Note 5 and Supplementary Fig. S4 ). In addition, on γ-79C-expressing oocytes, pre-treatment with the thiol-reactive compound methyl-(PEG) 11 -maleimide blocked the activity of subsequently applied MPC100 ( Supplementary Note 6 ). These findings indicate a dependence of MPC100 's persistent activity on tethering, specifically at the engineered cysteine site of the γ-79C receptor. Activity at GABA A Rs of retinal ganglion cells To test whether native neuronal GABA A Rs respond to MPC088 , we examined retinal ganglion cells (RGCs), a cell type known to abundantly express GABA A Rs [34] , [35] , [36] , [37] . When presented to single dissociated RGCs of rat retina, 10 μM trans -dominant MPC088 produced, on average, an approximately fivefold potentiation of the response elicited by 2 μM GABA, whereas cis -dominant MPC088 exhibited much less potentiation activity ( Fig. 5a ). At 30 μM, trans -dominant MPC088 alone produced a membrane current response whose peak amplitude amounted, on average, to 5% of the cell's response to 200 μM GABA ( Fig. 5b , inset). However, at 60 μM, the agonist effect increased to 43±9% of the response to 200 μM GABA ( n =7), and pre-treatment of trans -dominant MPC088 with UV light reduced this agonist activity by 88±6% ( n =4; P =0.002, two-sample Student's t -test; Fig. 5b ). Co-application of 100 μM PTX virtually eliminated the ganglion cell response to 2 μM GABA+10 μM trans -dominant MPC088 , and to 60 μM trans -dominant MPC088 alone ( Supplementary Note 7 and Supplementary Fig. S5 ), consistent with the mediation of trans - MPC088 's potentiation and direct activation by GABA A Rs. 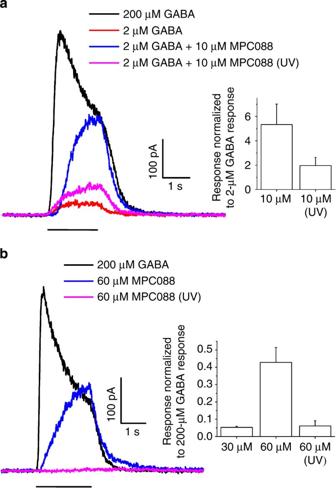Figure 5: Action ofMPC088on retinal ganglion cells. (a) Potentiation data obtained withtrans- andcis-dominant MPC088; thecis-dominant preparation was obtained by pre-treatingtrans-dominantMPC088with UV light for 5 min. Representative responses obtained from a single cell treated with 200 μM GABA (black), 2 μM GABA (red), 2 μM GABA co-applied with 10 μM oftrans-dominant (blue) orcis-dominant (magenta) MPC088. Inset: aggregate data (mean±s.d.) for potentiation factor determined withtrans- andcis-dominant MPC088 (left and right bars, respectively;n=6,P=0.003). (b) Direct activation data obtained withtrans- andcis-dominant MPC088. Representative responses obtained from a cell treated with 200 μM GABA (black), 60 μM oftrans-dominant (blue) and 60 μM ofcis-dominant (magenta) MPC088. Inset: aggregate data (mean±s.d.) for direct activation byMPC088. Left, middle and right bars show results obtained with 30 μMtrans-dominant (n=3), 60 μMtrans-dominant (n=7) and 60μMcis-dominant MPC088 (n=4), respectively. Figure 5: Action of MPC088 on retinal ganglion cells. ( a ) Potentiation data obtained with trans - and cis -dominant MPC088; the cis -dominant preparation was obtained by pre-treating trans -dominant MPC088 with UV light for 5 min. Representative responses obtained from a single cell treated with 200 μM GABA (black), 2 μM GABA (red), 2 μM GABA co-applied with 10 μM of trans -dominant (blue) or cis -dominant (magenta) MPC088. Inset: aggregate data (mean±s.d.) for potentiation factor determined with trans - and cis -dominant MPC088 (left and right bars, respectively; n =6, P =0.003). ( b ) Direct activation data obtained with trans - and cis -dominant MPC088. Representative responses obtained from a cell treated with 200 μM GABA (black), 60 μM of trans -dominant (blue) and 60 μM of cis -dominant (magenta) MPC088. Inset: aggregate data (mean±s.d.) for direct activation by MPC088 . Left, middle and right bars show results obtained with 30 μM trans -dominant ( n =3), 60 μM trans -dominant ( n =7) and 60μM cis -dominant MPC088 ( n =4), respectively. Full size image Photoregulation of GABA A Rs of cerebellar Purkinje neurons To evaluate the efficacy of MPC088 in GABA A R-expressing cells in situ , we conducted whole-cell voltage-clamp experiments on Purkinje neurons (PNs) in parasagittal slices from mouse cerebellum [38] , [39] ( Fig. 6 and Supplementary Methods ). PNs are known to express GABA A Rs of the α 1 β 2/3 γ 2 forms [26] , [27] , [28] . 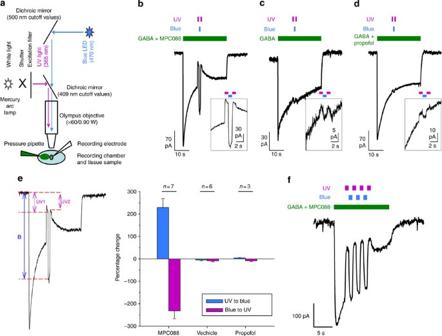Figure 6: Effect ofMPC088photoactivation on GABA-evoked currents in cerebellar PNs. (a) Optical configuration. (b) Representative trace from a whole-cell voltage-clamp recording from a PN. The cell was held at −70 mV, and 10 μM GABA+30 μMMPC088were applied via pressure pipette for 30 s. The cell was flashed with UV light (1 s, shuttered from a mercury arc lamp), then blue light (1 s, from a 470 nm LED) and then again with UV light (1 s). Insets expand the segments of the trace recorded when the light pulses were delivered. (c) Trace from the same cell as inb, but with exposure to 10 μM GABA alone. (d) Trace from the same cell as inb,c, but with exposure to 10 μM GABA+300 μM propofol. (e) Summary of results described inb–d. The left-hand trace shows the method used to obtain the numerical data shown at the right. The magnitude of the UV-to-blue transition was calculated as (B-UV1)/UV1; that of the blue-to-UV transition was calculated as (UV2-B)/UV2. Here, UV1, B and UV2 are, respectively, the magnitude of the current evoked by the first UV flash, the blue flash and the second UV flash, as referenced to the pre-GABA current level. The number above each condition indicates the number of cells from which data were obtained. For the negative control experiments (that is, those involving exposure to vehicle or propofol alone) in which no light-evoked current was detectable, current was measured for identical epochs at the terminations of the light pulses. Error bars represent the s.e.m. For both the blue-to-UV and the UV-to-blue transitions, the Kruskal–Wallis analysis of variance on ranks yieldedP<0.005 (H>11,df=2).Post-hocstatistical tests showed that results obtained withMPC088treatment differed significantly from those obtained under either negative control condition (Mann–Whitney rank-sum test:MPC088versus vehicle (blue-to-UV and UV-to-blue),P=0.002;MPC088versus propofol (blue-to-UV and UV-to-blue),P=0.014;P-values adjusted for multiple comparisons). (f) Representative trace from a cell exposed to multiple UV/blue light flashes during application of GABA andMPC088. Figure 6a shows the experimental setup, indicating how blue and UV light sources were combined in the epifluorescence pathway of an upright microscope. Currents were evoked in the PNs by applying 10 μM GABA from a local pressure pipette that also contained 30 μM trans -dominant MPC088 . UV illumination during the elicited response markedly decreased the membrane current; conversely, blue light enhanced the current ( Fig. 6b ). To determine whether these effects of light required the presence of MPC088 , we performed similar experiments on the same cell by replacing the pressure pipette with one that contained only GABA ( Fig. 6c ) or GABA plus propofol ( Fig. 6d ). By contrast with the Fig. 6b results, there was little or no light-induced current change under either condition. To quantify these results, we measured the current change in response to transitions from UV to blue light, and from blue to UV light ( Fig. 6e ). We found that the current changes produced by these transitions were opposite and, on average, equal in magnitude (mean ratio of absolute current magnitude in response to blue→UV/UV→blue was 1.00±0.01, a value that did not differ significantly from unity; P =0.86; one-sample Student's t -test, n =7; Fig. 6f ). Together, these results demonstrate that MPC088 directly modulates GABA A Rs of cerebellar PNs in situ. Figure 6: Effect of MPC088 photoactivation on GABA-evoked currents in cerebellar PNs. ( a ) Optical configuration. ( b ) Representative trace from a whole-cell voltage-clamp recording from a PN. The cell was held at −70 mV, and 10 μM GABA+30 μM MPC088 were applied via pressure pipette for 30 s. The cell was flashed with UV light (1 s, shuttered from a mercury arc lamp), then blue light (1 s, from a 470 nm LED) and then again with UV light (1 s). Insets expand the segments of the trace recorded when the light pulses were delivered. ( c ) Trace from the same cell as in b , but with exposure to 10 μM GABA alone. ( d ) Trace from the same cell as in b , c , but with exposure to 10 μM GABA+300 μM propofol. ( e ) Summary of results described in b – d . The left-hand trace shows the method used to obtain the numerical data shown at the right. The magnitude of the UV-to-blue transition was calculated as (B-UV1)/UV1; that of the blue-to-UV transition was calculated as (UV2-B)/UV2. Here, UV1, B and UV2 are, respectively, the magnitude of the current evoked by the first UV flash, the blue flash and the second UV flash, as referenced to the pre-GABA current level. The number above each condition indicates the number of cells from which data were obtained. For the negative control experiments (that is, those involving exposure to vehicle or propofol alone) in which no light-evoked current was detectable, current was measured for identical epochs at the terminations of the light pulses. Error bars represent the s.e.m. For both the blue-to-UV and the UV-to-blue transitions, the Kruskal–Wallis analysis of variance on ranks yielded P <0.005 ( H >11, df =2). Post-hoc statistical tests showed that results obtained with MPC088 treatment differed significantly from those obtained under either negative control condition (Mann–Whitney rank-sum test: MPC088 versus vehicle (blue-to-UV and UV-to-blue), P =0.002; MPC088 versus propofol (blue-to-UV and UV-to-blue), P =0.014; P -values adjusted for multiple comparisons). ( f ) Representative trace from a cell exposed to multiple UV/blue light flashes during application of GABA and MPC088 . Full size image We also examined the effects of MPC088 on action potential (AP) firing in PNs of the cerebellar slice. These experiments were similar to those described above, except that the cells were recorded under current-clamp to allow the cell to spike. To each of the PNs described in Fig. 7a,b , we first delivered GABA (10 μM) plus trans -dominant MPC088 (30 μM) by pressure application, and then exposed the cell to sequences of UV–blue–UV light. Exposure to GABA+ trans -dominant MPC088 decreased the firing rate by approximately 50%, on average ( Fig. 7b ). Furthermore, in all of the eight investigated cells, the UV–blue–UV flash sequence led to an increase, decrease and increase, respectively, in firing rate. Overall, the firing rate produced by blue light was 52±14% of that produced by UV light. In three of the eight PNs, blue light decreased the firing rate to <20% of that exhibited during the UV illumination, and one PN exhibited a blue-light-induced complete cessation of spiking that was reversed by subsequent UV light. As a negative control, we exposed cells to the UV–blue–UV light sequence, but in the absence of GABA/ MPC088 application. In these cells, there was no significant change in firing rate with any of the light flashes ( Fig. 7c ). Together, these data indicate a reversible, light-dependent action of MPC088 on PN spike-firing rate. 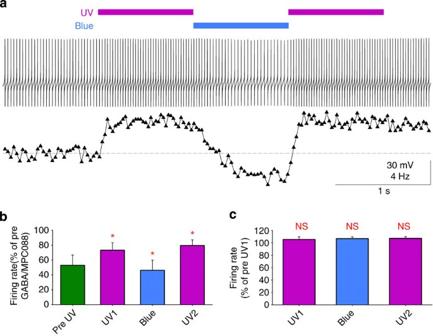Figure 7: Effect ofMPC088photoactivation on action potential firing frequency in PNs. (a) Representative data obtained by whole-cell current-clamp recording from a PN, which was injected with 468 pA to elicit a high-frequency train of action potentials. During this current step, 10 μM GABA+30 μMtrans-dominantMPC088were applied via pressure pipette for 10 s. The cell was then exposed for 1-s durations to UV light (UV1), then blue light, and then again with UV (UV2). The entire illustrated voltage versus time trace occurs during application of GABA/MPC088. Below this trace is plotted the instantaneous firing frequency versus time; the dashed line reflects the average firing frequency during the 1-s epoch that preceded the first UV exposure. (b) Summary of results from experiments of the type shown ina. Average spike frequencies were obtained for each cell in each of five 1-s epochs, then normalized to the pre-GABA/MPC088firing frequency (n=8 cells from 4 animals). Error bars here and increpresent the s.e.m. Repeated-measures analysis of variance on the aggregate data yieldedF(3,21)=10.213,P<0.001. Red asterisks above the purple and blue bars indicate significance of the average frequency in that epoch versus the preceding epoch (for example, the asterisk above the UV1 bar refers to significance of the average firing rate in the UV1 epoch versus the GABA/MPC088pre-UV epoch). Significance was determined frompost-hocpaired-sample Student'st-tests corrected for multiple comparisons, which yieldedP<0.02. (c) Summary of results from experiments similar to that described ina, but in which the cell was exposed only to the UV/blue/UV flash sequence (that is, no GABA/MPC088applied). Data normalized to the average firing frequency during the 1-s period preceding the first UV flash (n=7 cells from three animals). Repeated-measures analysis of variance on the aggregate data yieldedF(3,18)=3.057,P>0.05. Threepost-hocstatistical tests were then performed as described inb; none of these yielded significance at the uncorrected 0.05 level. Figure 7: Effect of MPC088 photoactivation on action potential firing frequency in PNs. ( a ) Representative data obtained by whole-cell current-clamp recording from a PN, which was injected with 468 pA to elicit a high-frequency train of action potentials. During this current step, 10 μM GABA+30 μM trans -dominant MPC088 were applied via pressure pipette for 10 s. The cell was then exposed for 1-s durations to UV light (UV1), then blue light, and then again with UV (UV2). The entire illustrated voltage versus time trace occurs during application of GABA/ MPC088 . Below this trace is plotted the instantaneous firing frequency versus time; the dashed line reflects the average firing frequency during the 1-s epoch that preceded the first UV exposure. ( b ) Summary of results from experiments of the type shown in a . Average spike frequencies were obtained for each cell in each of five 1-s epochs, then normalized to the pre-GABA/ MPC088 firing frequency ( n =8 cells from 4 animals). Error bars here and in c represent the s.e.m. Repeated-measures analysis of variance on the aggregate data yielded F (3,21)=10.213, P <0.001. Red asterisks above the purple and blue bars indicate significance of the average frequency in that epoch versus the preceding epoch (for example, the asterisk above the UV1 bar refers to significance of the average firing rate in the UV1 epoch versus the GABA/ MPC088 pre-UV epoch). Significance was determined from post-hoc paired-sample Student's t -tests corrected for multiple comparisons, which yielded P <0.02. ( c ) Summary of results from experiments similar to that described in a , but in which the cell was exposed only to the UV/blue/UV flash sequence (that is, no GABA/ MPC088 applied). Data normalized to the average firing frequency during the 1-s period preceding the first UV flash ( n =7 cells from three animals). Repeated-measures analysis of variance on the aggregate data yielded F (3,18)=3.057, P >0.05. Three post-hoc statistical tests were then performed as described in b ; none of these yielded significance at the uncorrected 0.05 level. Full size image To test for direct agonist activity of MPC088 on PNs, we perfused cerebellar slices with recirculating 30 μM MPC088 (the maximal MPC088 concentration we could reliably maintain solubilized in bicarbonate-buffered solution). MPC088 was converted to cis -dominant form by a 2-min exposure to UV light (light-emitting diode (LED), 365 nm, 160 mW, Mouser, Inc., Mansfield, TX, USA; LED driver, 700 mA BuckPuck DC Driver, Quadica Developments, Inc., Brantford, ON, Canada), before its dilution into the recirculating external solution. The same LED was then used to continuously UV-illuminate the recirculating solution for the duration of the experiment. We then obtained whole-cell voltage-clamp recordings from PNs and determined the change in membrane current produced by alternating blue and UV illumination of the slice, as in the Fig. 6 experiments. Of 44 cells examined, only 28 exhibited a current change >18 pA, which is the average amplitude of the blue-to-UV light currents from the vehicle and propofol conditions described in Fig. 6 . The average response from this subset of 28 cells was 80±13 pA. We then sought to test whether these currents were due to an agonist action of the drug, as opposed to a modulatory action occurring in concert with low levels of endogenous GABA present in the slice [40] . To discern modulation, we analysed the effect of added 30 μM gabazine [22] , [23] , a condition expected to inhibit the potentiating action of MPC088 (that is, to inhibit response enhancement dependent on endogenous GABA), but not to affect the direct agonist activity of MPC088 ( Fig. 2 ). In all but one of eight cells that exhibited light-evoked responses of >50 pA to the blue-to-UV switch, gabazine (30 μM) reduced the current to below the vehicle level of 18 pA ( Fig. 8a,b ). The average current remaining after gabazine treatment represented 11±3% of the pre-gabazine current ( Fig. 8b ). Even for the cell exhibiting the highest response of the 44 cells tested, gabazine completely abolished the response ( Fig. 8a ). Thus, at concentrations comparable to or lower than 30 μM, trans - MPC088 in cerebellar tissue is modulatory (endogenous GABA-dependent) rather than agonistic. 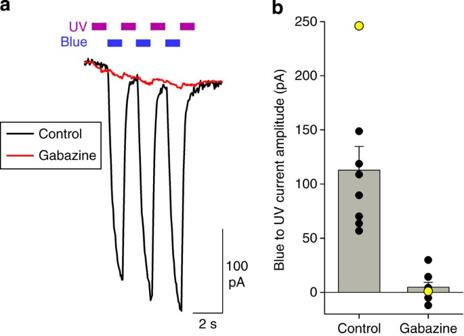Figure 8: Lack of agonist activity ofMPC088on PNs. (a) Averages of 10 recordings from a PN exposed to multiple blue/UV light flashes, in the presence ofcis-dominant MPC088 (30 μM) in the external solution, before (black) and after (red) the addition of gabazine (30 μM). There was no exogenous GABA present in the tissue. (b) Summary of results from eight experiments (eight PNs) including that described ina. The data indicate the magnitude of an outward current. The temporal sequence of illumination differed among the experiments (for example, only the cell inareceived multiple blue/UV exposures), but the data plotted are the amplitudes from the blue to UV transition (in the case of the cell ina, this is the blue/UV transition from the first of the three exposures). Yellow-filled data points indicate results from the experiment ina. Each data point is the average obtained from four to ten consecutive recordings. The light-evoked membrane current was significantly reduced by gabazine (Wilcoxon signed-rank test,P=0.008). Error bars represent the s.e.m. Figure 8: Lack of agonist activity of MPC088 on PNs. ( a ) Averages of 10 recordings from a PN exposed to multiple blue/UV light flashes, in the presence of cis -dominant MPC088 (30 μM) in the external solution, before (black) and after (red) the addition of gabazine (30 μM). There was no exogenous GABA present in the tissue. ( b ) Summary of results from eight experiments (eight PNs) including that described in a . The data indicate the magnitude of an outward current. The temporal sequence of illumination differed among the experiments (for example, only the cell in a received multiple blue/UV exposures), but the data plotted are the amplitudes from the blue to UV transition (in the case of the cell in a , this is the blue/UV transition from the first of the three exposures). Yellow-filled data points indicate results from the experiment in a . Each data point is the average obtained from four to ten consecutive recordings. The light-evoked membrane current was significantly reduced by gabazine (Wilcoxon signed-rank test, P =0.008). Error bars represent the s.e.m. Full size image Specificity of MPC088 for GABA A Rs on neurons To further address whether MPC088 has non-specific effects on excitability, we analysed the spikes elicited in the experiment described in Fig. 7 . We examined spikes recorded during exposure to GABA/ MPC088 ('puff') and under conditions in which MPC088 was absent, but in which the Purkinje cell received the UV–blue–UV light sequence ('no-puff'). The following three AP parameters were measured: peak amplitude, half width and maximum rise slope. Parameters were obtained from spikes occurring in the same 1-s epochs, in which average firing rate was significantly modulated by MPC088 (see Fig. 7b,c ). AP waveform parameters were calculated for pre-puff, blue light and UV epochs. Average values in the pre-treatment epochs for puff and no-puff did not significantly differ (spike amplitude (mV): 52±2 and 51±2; half width (ms): 0.61±0.03 and 0.57±0.03; maximum rise slope (mV ms −1 ): 150±10 and 161±13; P >0.4, unpaired Student's t -test). In addition, for each parameter, we normalized the average values for each cell and for each epoch to the averages in the pre-treatment epochs (pre-puff, pre-light). This analysis of excitability showed, first, that the only measurable effects on AP waveform are MPC088 -independent and caused by light exposure, and second, that the effect size of light is extremely small (less than 2%; Supplementary Fig. S6 and Supplementary Note 8 ). To test whether MPC088 affects excitatory synaptic transmission, we carried out whole-cell voltage-clamp recordings in CA1 pyramidal neurons of mouse hippocampus. As in the experiments of Fig. 8 , these recordings were obtained with perfusion of the slice with cis -dominant MPC088 (30 μM) under recirculation. PTX (100 μM) was also included in the external solution to block GABA A Rs. We evoked excitatory postsynaptic currents (EPSCs) by stimulating the Schaffer collaterals with a bipolar matrix microelectrode (FHC, Inc., Bowdoin, ME, USA), and recorded at a holding potential of +40 mV to uncover the NMDA receptor (NMDAR) component of the EPSC. We also presented paired electrical stimuli separated by 80 ms to assess possible effects of MPC088 on short-term plasticity. Each cell was given 20 interleaved trials in which the cell was exposed to two 0.1-s UV pulses surrounding a 1-s period of either blue light or no light ( Supplementary Fig. S7 and Supplementary Methods ). The effectiveness of the 0.1-s UV and the 1-s blue stimuli in photoconverting MPC088 was confirmed in separate experiments using 30 μM MPC088 and 3 μM GABA on the same preparation. To quantify the effects of MPC088 on AMPA receptors (AMPARs) and NMDARs, we measured, for the first EPSC of the pair, the peak current and the current just before the second stimulus, which reflect AMPAR and NMDAR components, respectively, of the EPSC [41] . Neither AMPAR-mediated nor NMDAR-mediated components of the EPSC were significantly altered by blue light ( Supplementary Fig. S7b ). In addition, blue light had no significant effect on the decay of the compound current (average τ from single-exponential fitting to the decay of the second EPSC: blue off, 131.2±11.1 ms; blue on, 130.9±11.3 ms; P =0.89, paired Student's t -test). There was also no significant effect of blue light on the paired-pulse ratio (measured as peak (second EPSC)/peak (first EPSC): blue off, 1.72±0.07; blue on, 1.85±0.14; P =0.34, paired Student's t -test). Together, these results indicate that MPC088 does not significantly affect presynaptic function, and that it has negligible actions on AMPAR-mediated and NMDAR-mediated EPSCs. The results demonstrate that MPC088 , a photoisomerizable compound derived from the allosteric ligand propofol, exerts a highly potent and light-sensitive regulation of GABA A Rs. Lights of differing wavelength can reversibly and in a quasi-stable manner interconvert the relatively active and inactive isomers of MPC088 ; this distinguishes the compound from a photosensitive ligand in which light activates the ligand by excitation of a fluorescent moiety [42] or by irreversibly eliminating a protective (caging) structural component. In addition to conferring pronounced light sensitivity to the receptor, MPC088 in its active ( trans ) form exhibits a potency considerably exceeding that of propofol itself. Our data indicate that the propofol moiety is required for activity, but it remains to be determined whether the high potency of MPC088 is due in addition to specific receptor-binding interactions with the butyryl, azobenzene and/or ethylenediamine moieties of the compound. Such a possibility is consistent with the finding that the α 1 β 3 (N265M)γ 2 GABA A R, which contains a substitution that strongly decreases the in vivo action of propofol [13] , exhibits reduced but still substantial sensitivity to trans - MPC088 . Furthermore, although the present results argue against a direct agonist action of trans - MPC088 on ligand-gated ion channels of cerebellar PNs other than GABA A Rs, the broad possibility remains that trans - MPC088 has physiological effects on non-GABA A R ion channels or other surface proteins of neural tissue. Particularly at higher concentrations, some broader activity of the compound would likely be tolerable, since propofol itself, while most active GABA A Rs [14] , is known to have effects on other cellular targets [43] . We have also examined the properties of MPC100 , a tetherable derivative of MPC088 that, via its terminating maleimide group, covalently binds to the cysteine-substituted γ-79C mutant form of the α 1 β 2 γ 2 GABA A R. The tethered compound exhibits persistent, light-regulated potentiating and activating effects on GABA A Rs. Thus, the tetherable MPC100 may have application in approaches that involve neuronal expression of a genetically engineered α 1 β 2 γ 2 GABA A R to which the photoswitch could be anchored, as in previous studies of potassium channels and L-glutamate receptors [15] , [17] , [19] . Furthermore, in contrast to previous structures designed for photocontrol of transmembrane ion channels [1] , [15] , [17] , [19] , a relatively long linear chain (PEG 24 ) separates the regulating structure ( MPC088 moiety) from the tethering moiety (maleimide). Beyond demonstrating that a long and flexible hydrophilic linker (and resultant high conformational entropy) can preserve substantial physiological activity of the distal MPC088 moiety, properties exhibited by MPC100 suggest the potential workability of other remote locations on the GABA A R itself for modulator attachment, or conjugation of the modulator to an affinity reagent designed for binding to the extracellular domain of the native GABA A R. As a general route to controlling neuronal activity with a modulating ligand, covalent binding of an introduced reactive (for example, maleimide-terminated) ligand to an engineered receptor site offers the advantage, in principle, of defining the precise receptor subtype [4] on which the ligand will act. However, this approach presents possible challenges relating to the need for inducing expression of the engineered receptor in the target cell type, and for avoiding problematic binding of the reactive ligand to unintended sites (for example, other cysteine-containing surface proteins) on both the target cells and others. The wide distribution of α 1 β 2 γ 2 GABA A Rs in the CNS tissues and the clinical importance of propofol encourage the investigation of MPC088 as a pharmacological tool in studies of CNS neural circuits. Toward this end, we have demonstrated that the compound reversibly modulates GABA currents in retinal neurons and cerebellar PNs, and that it can be used to reversibly control the spiking output of PNs. Given that PNs are intrinsically active at constant rates [38] , [39] , they are useful for examining this modulation because their spike rate gives a continuous readout of excitability. In providing the ability to control circuit excitability with spatial and temporal precision, switchable modulators of neural activity open new possibilities for exploring the links between neuronal activity and behaviour. For example, MPC088 and related diffusible compounds could allow regional induction of anaesthesia through the use of implanted optical fibres or a head-fixed preparation. This approach could be used to explore which brain regions are most important for anaesthesia and sedation. Clinical contexts in which a photoswitchable GABA A R modulator might be useful include diseases of hyperexcitability, such as epilepsy [44] , [45] , [46] , [47] . Propofol is known to be an effective therapeutic for intractable epilepsy, although side effects are a concern [48] , [49] , [50] . Photoswitchable propofol analogues, in combination with localized optical stimulation [51] and appropriate electrical monitoring, might enable a reduction of side effects in treating epilepsies, by employing spatially precise, optically regulated receptor modulation, specifically during bouts of hyperexcitability. Furthermore, even with a diffusible modulator, focally directed illumination could allow spatially restricted actions of the anti-epileptic drug around seizure foci. The photosensitivity and potency of MPC088 raise the possibility that compounds of this type might be used therapeutically in visual disorders. GABA A Rs are known to mediate visual signalling at multiple sites within the retina [34] , [35] , [37] , [52] , [53] , [54] ; GABA A Rs of retinal bipolar and ganglion cells are sensitive to propofol [55] , [56] ; and, as in oocytes expressing α 1 β 2 γ 2 GABA A Rs, responses of RGCs are potentiated and directly activated specifically by the trans -isomer of MPC088 ( Fig. 5 ). In diseases involving degeneration of the retina's rod and cone photoreceptors, MPC088 -inspired constructs of optimized wavelength sensitivity and relaxation kinetics [57] , and containing an affinity reagent-based anchor to provide cell-targeting specificity, may have application as a vision restoration therapy by establishing a photosensitivity of inner retinal neurons that effectively bypasses the dysfunctional rods and cones. Electrophysiological recordings Electrophysiological experiments were conducted on the following : (1) Xenopus laevis oocytes expressing GABA A Rs of defined subunit composition; (2) single, isolated ganglion cells of rat retina; (3) PNs in acute slice preparations of mouse cerebellum; and (4) CA1 neurons in acute slice preparations of mouse hippocampus. Animal care and all procedures involving the use of animals were conducted in accordance with institutional policies of the University of Illinois at Chicago (for Xenopus laevis and rats), and with the approval of the Chancellor's Animal Research Committee (Institutional Animal Care and Use Committee) at the University of California, Los Angeles (for mice). Xenopus laevis oocytes Oocytes expressing α 1 β 2 γ 2 receptors (rat α 1 , rat β 2 and human γ 2S ), α 1 β 3 γ 2 and α 1 β 3 (N265M)γ 2 (rat β 3 and β 3 (N265M)), and α 4 β 3 δ (rat α 4 and δ) were prepared and studied by two-electrode voltage-clamp recording [58] (holding potential: −70 mV; amplifier: GeneClamp500B, Axon Instruments, Foster City, CA, USA). Unless otherwise indicated, oocytes were superfused with Ringer solution (physiological saline) at a rate of ~1 ml min −1 . The experiments of Figs 1d,e and 2c–e , and Supplementary Figure S4 involved periods of static bathing, that is, halted superfusion. The γ 2 (A79C) subunit was prepared by site-directed mutagenesis. Oocyte electrophysiological experiments were carried out in room light. A UV-LED (peak wavelength: 365 nm; Hamamatsu Photonics, Japan) and a microscope illuminator (white light; Schott Fostec, Auburn, NY, USA) provided UV and visible stimulating light. As measured at the position of the oocyte, the intensity of the UV light at 365 nm was 220 μW mm −2 . At 440 nm, the nominal strength of the visible (white) light (referred to as high-intensity visible light) was 28 μW mm −2 and that of the ambient room illumination was 0.045 μW mm −2 . In all experiments, low-intensity visible light from the microscope illuminator (3 μW mm −2 at 440 nm) was present at all times, except those involving high-intensity visible illumination. Electrophysiological data were obtained using Clampex 8.2 (Axon Instruments) and analysed using Clampfit 10.0 (Axon Instruments) and OriginPro7.5 (OriginLab, Northampton, MA, USA). RGCs of rat Experiments were conducted on enzymatically dissociated ganglion cells obtained from adult Sprague-Dawley rats (male and female, 6–16 weeks of age; Charles River Laboratories, Wilmington, MA, USA). Procedures for killing, isolation of the retina and the dissociation of retinal cells were as described previously [59] , except that the period of retinal cell dissociation was shortened from 40 to 20 min. Isolated ganglion cells were identified on the basis of their morphological appearance and the presence of a large voltage-gated sodium current. Whole-cell patch-clamp techniques similar to those described [59] were used to record membrane current responses to test agents. The patch pipette with a resistance of 8–12 MΩ was pulled in two stages using a micro-electrode puller (Model PP830, Narishige Group, Tokyo, Japan). The pipette was filled with an intracellular solution containing 95 mM CsCH 3 SO 3 , 20 mM TEA-Cl, 10 mM glutamic acid, 1 mM BAPTA, 10 mM HEPES, 8 mM phosphocreatine di(tris), 1 mM MgATP and 0.2 mM Na 2 GTP; pH adjusted to 7.2 with CsOH. Cells were clamped at 0 mV (Axopatch 200B amplifier, Axon Instruments), and experimental runs were controlled by pCLAMP system software (Axon Instruments). Electrophysiological data were obtained in response to test compounds dissolved in physiological saline (Ringer solution) that consisted of 135 mM NaCl, 5 mM KCl, 2 mM CaCl 2 , 2 mM MgCl 2 , 10 mM glucose and 5 mM HEPES, pH 7.4. Supplementation of aqueous test solutions with MPC088 was carried out by adding an aliquot of a stock solution containing the compound dissolved in dimethyl sulfoxide. In all experiments, the amount of carrier dimethyl sulfoxide present in the applied test solution was <1% (v/v). Test solutions were delivered from separate reservoirs by a multi-channel perfusion system. The same UV–LED used in the oocyte experiments was used for UV illumination of MPC088 -supplemented test solutions. For preparation of cis -dominant MPC088, the test solution of initially trans -dominant compound underwent a 5-min UV illumination before its placement in the perfusion reservoir. All preparative procedures were performed in the dark, and the reservoirs and perfusion lines were light-protected with aluminium foil. As in the oocyte experiments, data were analysed with Clampfit and plotted with Origin. Unless otherwise stated, numerical data from replicate experiments are presented as mean±s.d., and all statistical analyses of data obtained from oocytes and from RGCs employed a two-sample Student's t -test. Cerebellar PNs from mice Experiments on cerebellar PNs employed acute slices obtained from cerebella of 16- to 30-day-old C57/BL6 mice (Charles River Laboratories). After induction of deep anaesthesia with isoflurane, mice were decapitated, and the cerebellum vermis was removed and placed in an ice-cold cutting solution containing (in mM): 85 NaCl, 2.5 KCl, 0.5 CaCl 2 , 4 MgCl 2 , 1.25 NaH 2 PO 4 , 24 NaHCO 3 , 25 glucose and 75 sucrose. A Leica VT1000 vibratome was used to cut 250-μm thick, sagittal slices from the cerebellar vermis. Slices were then placed in an external recording solution containing (in mM): 119 NaCl, 2.5 KCl, 2 CaCl 2 , 1 MgCl 2 , 1 NaH 2 PO 4 , 26.2 NaHCO 3 and 25 glucose. The solution was warmed to 35 °C for 15–20 min and then allowed to reach room temperature. Both the cutting solution and the recording solution were continuously bubbled with 95% O 2 /5% CO 2 , and the recording solution was perfused at the rate of 2–4 ml min −1 . Whole-cell voltage-clamp recordings were carried out at room temperature from PNs with an Axopatch 200A amplifier (Axon Instruments) and the neurons were held at −70 mV. Recording pipettes had bath resistances of 2–6 MΩ and were pulled using a horizontal micropipette puller (Model P-1000 Flaming/Brown Micropipette Puller, Sutter Instrument Company, Novato, CA, USA). The internal solution for voltage clamp ( Figs 6 and 8 ) contained (in mM): 140 CsCl, 3 NaCl, 10 HEPES, 2 MgCl 2 , 4 ATP, 0.4 GTP, 1 EGTA, 10 TEA-Cl and 5 QX-314 Br (to block respectively, K v and Na v channels), and pH was adjusted to 7.4 with CsOH. Cs-based internal solutions prevented a small, UV light-elicited, transient outward current that was seen in the absence of GABA or MPC088 . In some recordings, CdCl 2 (100 μM) was included in the external solution to block synaptic transmission. Although we found no differences in the magnitudes of the MPC088 -dependent currents, this had two benefits; it reduced spontaneous synaptic activity, which would otherwise appear as high frequency noise on the traces, and it confirmed that MPC088 actions were cell-autonomous. Whole-cell current-clamp recordings from PNs were carried out at room temperature with the same equipment as described above. Recording pipettes had bath resistances of 6–9 MΩ. The internal solution substituted 126–130 mM KMeSO 3 for CsCl/(TEA-Cl) and contained 5 mM EGTA. In some cases, internal solutions for current clamp included 5 mM phosphocreatine and KCl substituted for NaCl to yield a final chloride concentration of 14 mM. Where appropriate, distilled water was added to adjust final osmolarity. In some cases, positive current was injected into the PNs to elicit spiking. Local drug application to the PNs was achieved with a glass pipette (2–3 μm tip diameter) filled with the solution containing the indicated compounds dissolved in filtered external recording solution. Pressure pulses (0.5 to 2 psi) were provided by a Picospritzer II (Parker Hannifin Co., Cleveland, OH, USA). Data from cells were excluded from analysis if there was no detectable decrease in firing rate with GABA+ MPC088 application. They were also excluded if the average baseline (2-s epoch before drug application) firing rates fell outside the range 5 to 100 Hz, or if the cell stopped firing completely in the midst of the trial and did not recover by the end of the trial. Pulses of UV light were presented to the tissue by shuttering a 100 W mercury arc lamp. Light from this source was collimated and focused through the objective lens of the recording apparatus. The broad-spectrum light from the arc lamp passed through an excitation filter (366 nm; full-width at half-maximum, 16.6 nm; Semrock, Inc., Rochester, NY, USA) to isolate the UV component, and reflected off a dichroic mirror (409 nm cutoff wavelength, Semrock, Inc.; Fig. 6a ). The blue light source was a 470 nm LED (Quadica Developments, Inc.) that was connected to a beamsplitter cube (Siskiyou Designs, Grants Pass, OR, USA) located in the infinity space above the objective. The blue light was reflected by the dichroic mirror (500 nm cutoff wavelength, Chroma Technology Co., Bellows Falls, VT, USA) positioned in the beamsplitter cube such that it passed through the 409-nm dichroic mirror in the UV filter cube to reach the slice. This configuration allowed UV and blue light to be combined in the epifluorescence path and to be independently controlled. To minimize exposure of the slice preparation and MPC088 -containing solutions to ambient room light, the experimental apparatus housing the cerebellar slice, microscope, micro-manipulators and perfusion lines was shielded by a dark curtain, and a photographic safe light was used inside the area housing these components. Illumination from the microscope lamp used for visual inspection of the tissue passed through a Wratten 2 29 filter that attenuated wavelengths below 600 nm. All data from experiments on PNs are presented as mean±s.e.m. How to cite this article: Yue, L. et al . Robust photoregulation of GABA A receptors by allosteric modulation with a propofol analogue. Nat. Commun. 3:1095 doi: 10.1038/ncomms2094 (2012).